Turning a band insulator into an exotic superconductor Understanding exotic, non- s -wave-like states of Cooper pairs is important and may lead to new superconductors with higher critical temperatures and novel properties. Their existence is known to be possible but has always been thought to be associated with non-traditional mechanisms of superconductivity where electronic correlations play an important role. Here we use a first principles linear response calculation to show that in doped Bi 2 Se 3 an unconventional p -wave-like state can be favoured via a conventional phonon-mediated mechanism, as driven by an unusual, almost singular behaviour of the electron–phonon interaction at long wavelengths. This may provide a new platform for our understanding of superconductivity phenomena in doped band insulators. Since Bardeen, Cooper and Schrieffer’s (BCS) seminal discovery of their microscopic theory of superconductivity in 1957 (ref. 1 ), there has been more than a half-century work to understand how the Cooper pairs can condense into the states with the angular momentum greater than spherically symmetric s -state of the BCS theory. Such possibilities in much celebrated heavy fermion [2] and high- T c (critical temperature ) cuprate superconductors [3] , Sr 2 RuO 4 (ref. 4 ) and superfluid He 3 (ref. 5 ) are widely known but have nothing to do with the original BCS idea that elementary excitations of the lattice, phonons, are responsible for the formation of the Cooper pairs, and, despite a great amount of discussion [6] , [7] , [8] , [9] , [10] , [11] , [12] , there is no well-accepted example that the phonon-mediated unconventional pairing is indeed realized in nature. A recently triggered search for novel topological superconductors [13] , [14] , [15] , [16] has, however, raised this issue to a completely new level with some revolutionary promising applications for fault-tolerant quantum computing [17] . Here we demonstrate that some doped band insulators with layered structures and strong spin–orbit coupling where time reversal and inversion symmetries are unbroken can be good candidate materials in realizing an unconventional state of the fermions pair that are attracted via conventional phonon-mediated mechanism. We address this problem by performing first principle density-functional linear response calculations [18] of full wave–vector-dependent electron–phonon interaction (EPI) in doped band insulator Bi 2 Se 3 and argue that a highly unusual case of a singular coupling is realized for this material. We discuss the consequences of such singular behaviours and uncover which peculiar details of the electrons interacting with lattice can provide a novel platform for unconventional superconductivity phenomena. Our numerical results are presented for the archetypal topological insulator Bi 2 Se 3 (ref. 19 ), but the characteristic features of its bulk spectrum of electrons as well as their interactions with lattice are expected to be generic for other systems, not related to their topological aspect. Our findings include: (1) very large electron–phonon matrix elements in the long-wavelength limit for those vibrational modes that break the inversion symmetry and lift the band degeneracy of strongly spin–orbit-coupled Fermi electrons; (2) a very large contribution to the electron–phonon coupling constant λ from the acoustic phonons due to their low vibrational frequencies; (3) a strong Fermi surface (FS) nesting at small wavevectors q along the z -direction due to layered nature of the lattice that enhances λ . Our calculated coupling constants for all s , p and d pairing channels are found to be very close to each other. By further considering the effects of the Coulomb pseudopotential μ * and some spin–fluctuation-induced interaction, we propose that pairs with higher angular momentum are favoured in doped Bi 2 Se 3 and it may be the first phonon-mediated unconventional superconductor with the A 2 u symmetry ( p z -like nodal pseudospin triplet) of its order parameter. Singular EPI model A solution for the superconducting critical temperature T c in a given α-pairing channel is described by the BCS formula T c,α =1.14 ω D exp[−1/ λ α ] where ω D is the Debye frequency and the electron–phonon coupling constant λ α is given by the FS average of the EPI W ( k , k ′): Here ɛ k and N (0) are the energies and density of states of the electrons with respect to the Fermi level, while η α ( k ) represents a set of orthogonal FS polynomials, ∑ k η α ( k ) η β ( k ) δ ( ɛ k )/ N (0)= δ αβ , such as crystal [20] or FS [21] harmonics introduced as generalizations of spherical harmonics for arbitrary surfaces. In the original BCS limit, W ( k , k ′) is just a constant that automatically produces λ α =0 for all α > s due to the orthogonality of η α ( k ). In reality, W ( k , k ′) is a slow-varying function of k and k ′, which makes the coupling constant λ with α = s largest among all possible pairing channels and results in a largest energy gain by forming the pairs of the s -wave symmetry for practically all known electron–phonon superconductors. Instead of a weakly momentum-dependent EPI, let us imagine an extreme case of a singular coupling at only certain wavevector q 0 (together with its symmetry-related partners). Namely, assume that W ( k , k ′) ≃ W 0 δ ( k − k′ − q 0 )= W 0 ∑ α η α ( k ) η α ( k′ + q 0 ). Then λ α = W 0 ∑ k η α ( k ) η α ( k + q 0 ) δ ( ɛ k ). It is then clear that the overlap between any two α> s polynomials separated by q 0 is always smaller than the one for η s ( k )≡1 and the s -wave pairing still wins. This is unless q 0 →0, or if the original FS and the one shifted by q 0 are indistinguishable, in which cases all pairing channels become degenerate and compete with each other. This provides us with a general idea where to find unconventional superconductors with conventional electron–phonon mechanism. In particular, we argue by our first principles linear response calculation [18] that this exact case of a singular EPI with strongly nested FS at long wavelengths is realized for Cu x Bi 2 Se 3 . Relevance to topological superconductivity Our study has a direct relevance to the search of novel topological superconductors requiring an odd parity fully gapped state of Cooper pairs [22] that have recently attracted a great interest due to the existence of Majorana modes that appear inside a superconducting energy gap [13] . Such exotic states are traditionally thought to be associated with an electronic mechanism of superconductivity, but the proposed candidate materials, such as Cu x Bi 2 Se 3 (ref. 23 ), TlBiTe 2 (ref. 24 ) and Sn 1− x In x Te (ref. 25 ), are systems with weakly correlated sp electrons [23] , [24] , [25] , and it is likely that the conventional phonon-mediated mechanism plays a major role. There are currently hot debates in the literature about the pairing symmetry in Cu x Bi 2 Se 3 (refs 22 , 23 , 26 , 27 , 28 , 29 , 30 ): based on a two-orbital model, Fu and Berg [22] proposed that it is a topological superconductor with a fully gapped state of odd parity pairing. Using tunnelling experiments, two groups have observed zero-bias conductance peak, which may be a signature of topological surface states associated with non-trivial pairing [27] , [28] . The absence of the Pauli limit and the comparison of critical field B c2 ( T ) to a polar-state function indicates a spin–triplet superconductivity [29] . However, contrary to these viewpoints, a recent scanning tunnelling microscopy measurement suggests that Cu 0.2 Bi 2 Se 3 is a classical s -wave superconductor with a momentum-independent order parameter [30] . At the absence of any other examples in nature that phonons can trigger a pairing state other than s , does this experiment provide a most plausible scenario for this highly interesting phenomenon? Since Cu x Bi 2 Se 3 crystals are intrinsically inhomogeneous, it may be difficult to elucidate the features of the mechanism as mentioned above. And very recently, it was found that under high pressure, Bi 2 Se 3 displays anomalous superconducting behaviour indicating the unconventional pairing [31] . Linear response calculations of phonons and their linewidths Here we apply density functional linear response method to study the problem of doped Bi 2 Se 3 . Our numerical electronic structures are in accord with previous theoretical results [19] . Our calculated phonon dispersions for Bi 2 Se 3 along several high-symmetry directions of the Brillouin zone (BZ) are shown in Fig. 1 , where similar to prior work [32] , we see that the phonon frequencies of Bi 2 Se 3 span up to 5.5 THz, and all vibrational modes are found to be quite dispersive despite its two-dimensional-like layered structure. There are two basic panels in the phonon spectrum: the top nine branches above 2.5 THz are mainly contributed by vibrations of Se atoms, while the six low branches come from the Bi modes. Our calculated phonon frequencies at Γ agree with the experimental [33] , [34] and previous numerical results [32] very well. 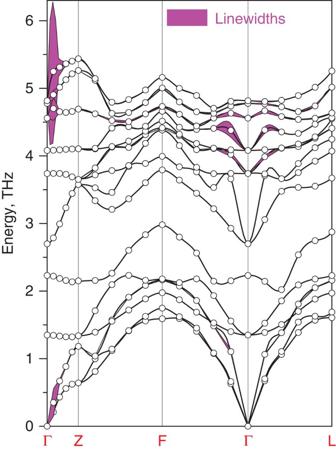Figure 1: Description of lattice dynamical properties. Calculated phonon dispersions (points) of Bi2Se3using density-functional linear response approach. The widening shows our caclulated phonon linewidth arising from the EPI in CuxBi2O3(x=0.16). Figure 1: Description of lattice dynamical properties. Calculated phonon dispersions (points) of Bi 2 Se 3 using density-functional linear response approach. The widening shows our caclulated phonon linewidth arising from the EPI in Cu x Bi 2 O 3 (x=0.16). Full size image It is found that superconducting Cu x Bi 2 Se 3 has the maximum T c of 3.8 K at x ~0.12 (ref. 23 ) and on further doping the T c gradually decreases, but superconductivity remains till x ~0.6 (ref. 26 ). The copper atoms populate into the interlayer gaps [23] and have a small effect on the structural properties [34] , [35] . To simulate the doping, we perform virtual crystal approximation calculation with adding x electrons into the unit cell as a uniform background and calculate wavevector ( q )- and vibrational mode (ν)-dependent phonon linewidths γ q ν from which the electron–phonon coupling constant can be deduced [36] . Our calculated phonon linewidths γ q γ for a representative doping x =0.16 are shown in Fig. 1 by widening the phonon dispersion curves ω q ν proportionally to γ q γ . A striking feature is that only the phonons along ΓZ line of the BZ, especially one optical mode with the vector q =(0,0,0.04)(2π)/( c ) has a very large linewidth. We also note a considerable linewidth for a longitudinal acoustic mode at the same q . This is in principle detectable via neutron-scattering experiment. Interestingly, as the contribution to λ from each mode is proportional to γ q ν divided by , it is the acoustic mode that would provide a dominant contribution to total λ rather than the optical one. Origin of large EPI We first look at possible nesting like features of the FS. We mark time reversal invariant momenta (Γ(000), L(π,0,0), F(π,π,0) and Z(π,π,π)) of the first BZ in Fig. 2a , and show our calculated FS for x =0.16 in Fig. 2b that is open, in agreement with recent ARPES and dHvA measurements [37] . Although the FS has strong three-dimensional features, there is a prism-like electron pocket around the Γ point that indicates a nesting for the wavevectors along the Γ Z line. To confirm this result, Fig. 3a shows our calculated nesting function X ( q )=∑ k δ ( ɛ k ) δ ( ɛ k + q ) within the plane that contains ΓFZL points of the BZ. One can see clearly that X ( q ) exhibits a ridge along the ΓZ line, where the nesting function reaches its largest values as q approaches zero along Γ Z . This is despite a general tendency for X ( q ) to diverge as q →0, that is connected to a commonly used linearization of imaginary electronic susceptibility Im χ( q , ω ) with respect to ω when it is within the range of the phonon frequencies; the approximation that breaks down for small wave vectors but is irrelevant for estimating any types of three-dimensional integrals over q due to the appearance of the q 2 prefactor. 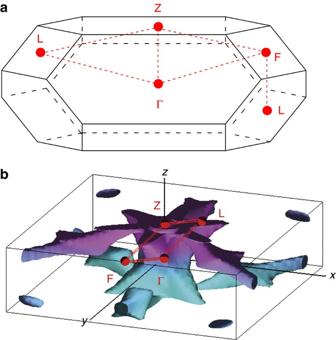Figure 2: Calculation for the FS. (a) BZ of hexagonal Bi2Se3where we mark the time reversal invariant momenta Γ(000), L(π,0,0), F(π,π,0) and Z(π,π,π). (b) FS of CuxBi2Se3for dopingx=0.16. A colour (magenta positive, cyan negative) corresponds to a proposedp-wave solution for the superconducting energy gap of theA2usymmetry discussed in text. Figure 2: Calculation for the FS. ( a ) BZ of hexagonal Bi 2 Se 3 where we mark the time reversal invariant momenta Γ(000), L(π,0,0), F(π,π,0) and Z(π,π,π). ( b ) FS of Cu x Bi 2 Se 3 for doping x =0.16. A colour (magenta positive, cyan negative) corresponds to a proposed p -wave solution for the superconducting energy gap of the A 2 u symmetry discussed in text. 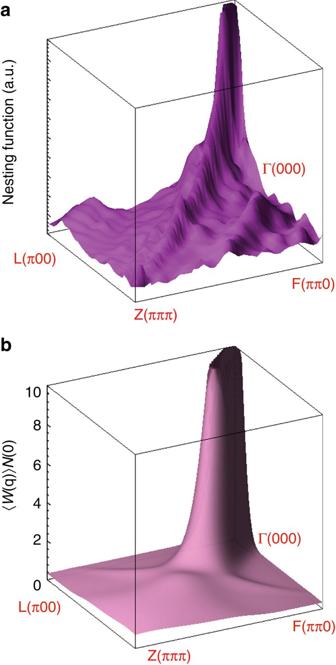Figure 3: Behaviour of the electron–phonon pairing interaction. (a) Calculated nesting function for CuxBi2Se3corresponding tox=0.16. Notice that the basal area given by ΓFZL points of the momentum space is in fact rhombus as seen from the BZ plot shown inFig. 2a. (b) Calculated average electron–phonon pairing interaction ‹W(q)›N(0) as a function of momentum within the basal area ΓFZL. Full size image Figure 3: Behaviour of the electron–phonon pairing interaction. ( a ) Calculated nesting function for Cu x Bi 2 Se 3 corresponding to x =0.16. Notice that the basal area given by ΓFZL points of the momentum space is in fact rhombus as seen from the BZ plot shown in Fig. 2a . ( b ) Calculated average electron–phonon pairing interaction ‹ W ( q )› N (0) as a function of momentum within the basal area ΓFZL. Full size image A strong enhancement of the electron–phonon coupling due to nesting is an interesting but not an uncommon effect in metals. In particular, nesting alone will not result in any type of unconventional pairing, as the latter is the property of the peculiar behaviour of the pairing interaction W ( k , k ′) appeared in equation (1). To analyse it, we introduce the following average The plot of ‹ W ( q )› N (0)) within the ΓFZL plane is shown in Fig. 3b . Remarkably, we again find a strongly enhanced function that is peaked at small values of q once it approaches zero along Γ Z . As all nesting features have been eliminated, it is interesting to understand the nature of this highly non-trivial behaviour that originated from the acoustic and the optical modes. Both essentially correspond to the motion of the Bi atoms along z -direction. By ignoring the smallness of the wave vector, we performed the calculation for q =0 by moving the atoms according to the eigenvectors of the optical mode. Such deformation potential calculation is shown in Fig. 4 where the band structures for the undistorted ( Fig. 4a ), and the distorted ( Fig. 4b ) lattices are plotted in the vicinity of the Fermi level to illustrate the crucial change in the electronic structure. Bi 2 Se 3 has both time-reversal symmetry and the inversion symmetry, and despite the presence of spin–orbit coupling, this results in every energy band to be at least double degenerate for the undistorted structure. The discussed phonon displacement breaks the inversion symmetry and lifts the double degeneracy, resulting in a large EPI. It is worth to mention that this effect only exists for the system with both inversion symmetry and strong spin–orbit coupling, and the spin–orbit coupling is essential here but in its very unusual role to generate a large EPI. In addition to this effect, there is a considerable renormalization of the bandwidth as well as other noticeable features as illustrated in Fig. 4 that result in the strongly enhanced EPI at long wavelengths. 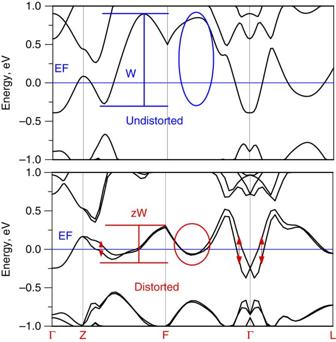Figure 4: Illustration of large coupling by deformation potentials. Calcuated energy bands for the undistorted (a) and distorted (b) structures of Bi2Se3, corresponding to the Γ point optical mode associated with the inversion breaking dispacement of Bi atom alongz-axis. Illustrated are the splitting of double degenerate bands as well as renormalization of their width that result in a large EPI. Figure 4: Illustration of large coupling by deformation potentials. Calcuated energy bands for the undistorted ( a ) and distorted ( b ) structures of Bi 2 Se 3 , corresponding to the Γ point optical mode associated with the inversion breaking dispacement of Bi atom along z -axis. Illustrated are the splitting of double degenerate bands as well as renormalization of their width that result in a large EPI. Full size image Results for electron–phonon coupling constants We now discuss our calculated total values of the electron–phonon λ α for various pairing channels that are classified according to the D 3 d point group of Bi 2 Se 3 . Since here the single-particle states are affected by spin–orbit coupling, the Cooper pairs are no longer pure spin singlets or triplets but should be composed from superpositions of spinor states. However, the presence of time reversal and inversion symmetries ensures the twofold degeneracy of the Fermi electrons (conveniently labelled via the use of a pseudospin index) from which the Cooper pairs of even/odd parity and of zero momentum are composed [38] . We use crystal harmonics for the FS polynomials after ref. 20 . For a representative doping with x =0.16 we obtain =0.45 ( s -like) for the even parity pseudospin singlet, and =0.21 ( p x / y -like), =0.39 ( p z -like) for the odd parity pseudospin triplets. We also evaluated the coupling constants with d -wave-like symmetries and obtained the values of λ around 0.2 for the two E g symmetries and 0.37 for the A 1 g ( ) one. Consistent with the discussion of our singular electron–phonon model, one can see a remarkable proximity of all pairing constants, and especially of . Very similar trends hold for slightly smaller and larger values of x where we find that all couplings constants change monotonically with doping. Finally, we note that the effective coupling should include the effect of the Coulomb pseudopotential μ * and other possible renormalizations such as, for example, spin fluctuations. It is well known that the values of μ s * range between 0.10 and 0.15 for most s -wave electron–phonon superconductors. We also expect that for the pairings with higher angular momentum [11] . While we do not expect that spin fluctuations are essential for the sp electron material like doped Bi 2 Se 3 , we have also evaluated spin fluctuational λ s using a single-band fluctuation exchange approximation [39] . Using a representative value of U =0.5 eV (which approximately constitutes 0.4 of the electronic bandwidth) we have obtained for x =0.16: , which produces slightly negative (repulsive) contributions for the s - and d -wave and slightly positive (attractive) ones for the p -wave pairings. Overall, combining these data in the effective coupling , we see that it favours the pseudotriplet pairing of A 2 u symmetry in doped topological superconductor Bi 2 Se 3 , and is capable of producing the values of T c =3~5 K. The behaviour of the superconducting energy gap for this symmetry is shown by colouring the FS in Fig. 2b , where the nodal plane corresponds to k z =0. Calculations for other systems In addition to doped Bi 2 Se 3 , we also performed similar studies for TlBiTe 2 (ref. 24 ) and Sn 1− x In x Te (ref. 25 ). For both compounds, in a wide range of carrier concentration, we cannot find any singular behaviour of EPI, and our results show that the coupling in s -wave pairing channel is considerably larger than that in all other channels. Thus we believe that TlBiTe 2 and Sn 1− x In x Te are conventional s -wave superconductors. In perspective, we think that our discussed effects could be present in several other layered band insulators where strong spin–orbit coupling as well as unbroken time reversal and inversion symmetries could interplay with certain lattice distortions and create exotic superconducting states upon doping. Synthesizing such systems with isolating their thin flakes using a famous graphene’s scotch tape method should not be too difficult to make. This may provide a new platform for realizing unconventional superconductivity in general. Although our proposed solution for Bi 2 Se 3 is gapless pseudospin triplet, an odd-parity fully gapped pairing state thought in a topological superconductor can also in principle be realized in other systems using the above-discussed singular EPI. Finally, a gate tuning was recently used to introduce a carrier doping in monolayered MoS 2 and turned on superconductivity [40] , which may be a good way to overcome the inhomogenuity in Cu x Bi 2 Se 3 and experimentally clarify the nature of its pairing state. The results reported here were obtained from density functional linear response approach, which has been proven to be very successful in the past to describe EPIs and superconductivity in metals [41] , including its applications to plutonium [42] , MgB 2 (ref. 43 ), lithium-deposited graphene [44] and many other systems [45] . The full potential all-electron linear–muffin–tin–orbital method [18] had been used, and an effective (40,40,40) grid in k -space (total 10,682 irreducible k points) has been used to generate γ q γ on (6,6,6), (8,8,8) and (10,10,10) grids of the phonon wavevector to ensure the convergence of the calculated results. How to cite this article: Wan, X. & Savrasov, S. Y. Turning a band insulator into an exotic superconductor. Nat. Commun. 5:4144 doi: 10.1038/ncomms5144 (2014).